Ultralow viscosity of carbonate melts at high pressures Knowledge of the occurrence and mobility of carbonate-rich melts in the Earth’s mantle is important for understanding the deep carbon cycle and related geochemical and geophysical processes. However, our understanding of the mobility of carbonate-rich melts remains poor. Here we report viscosities of carbonate melts up to 6.2 GPa using a newly developed technique of ultrafast synchrotron X-ray imaging. These carbonate melts display ultralow viscosities, much lower than previously thought, in the range of 0.006–0.010 Pa s, which are ~2 to 3 orders of magnitude lower than those of basaltic melts in the upper mantle. As a result, the mobility of carbonate melts (defined as the ratio of melt-solid density contrast to melt viscosity) is ~2 to 3 orders of magnitude higher than that of basaltic melts. Such high mobility has significant influence on several magmatic processes, such as fast melt migration and effective melt extraction beneath mid-ocean ridges. Carbonate-rich magmas are rarely erupted at the Earth's surface, but are important to Earth’s magmatism at depth. Carbonatite is an igneous rock containing >50% magmatic carbonate minerals that occurs on all continents, from the Archean to the present day [1] , and derives from carbonate-rich magmas in the upper mantle [2] , [3] , [4] . Kimberlite is another carbonate-rich magma, typically intruded into the crust of ancient and stable cratons [5] , [6] , [7] . Kimberlite magma is characterized by low silica with high magnesium and a C–O–H volatile-rich composition [5] , [6] , [7] , [8] , and is thought to be formed in the presence of H 2 O and CO 2 under conditions close to the carbonate–peridotite solidus in the Earth’s mantle [9] , [10] , [11] . Small amounts of carbonate-rich melt may also be present in the asthenosphere beneath mid-ocean ridges, according to recent electrical conductivity studies [12] , [13] and high-pressure and high-temperature experiments [10] , [14] , [15] , [16] . In addition, strongly carbonated silicate melt is thought to be partly responsible for the presence of oceanic low-velocity zones [10] , [17] . Despite extensive studies on the occurrence and stability of carbonate-rich melts, physical properties (such as density, viscosity and mobility) of carbonate melts have not been well-understood. Viscosity is one of the most important transport properties controlling migration processes of melts in the Earth’s interior [18] . Viscosities of numerous silicate, oxide and metallic melts have been investigated by falling-sphere viscometry at high-pressure conditions [19] , [20] , [21] , [22] , [23] , [24] , [25] . By contrast, there are only limited experimental data on the viscosity of carbonate at high pressures and temperatures. One study reported viscosity of a melt with 70 wt.% CaCO 3 and 30 wt.% MgCO 3 at 1 GPa (ref. 26 ) by ex situ falling-sphere viscometry, based on examination of probing sphere positions in quenched samples. The viscosity values thus obtained, 5.7 Pa s at 1,200 °C and 0.8 Pa s at 1,300 °C, are associated with large uncertainties. An in-situ viscosity measurement using synchrotron X-ray radiography was carried out for potassium carbonate melts (K 2 Mg(CO 3 ) 2 and K 2 Ca(CO 3 ) 2 ) in ref. 27 . However, because K 2 Mg(CO 3 ) 2 has a structure distinct from other carbonate melts as evidenced by glass formation on quenching [28] , it likely does not represent typical carbonate melts. In addition, the frame rate employed for capturing images of the falling sphere during these experiments was insufficient to accurately define the terminal velocity, which is the basis for viscosity determination. Here we investigate viscosities of liquid calcite (CaCO 3 ) and natural dolomite ((Mg 0.40 Fe 0.09 Ca 0.51 )CO 3 ) up to 6.2 GPa using an advanced technique of viscosity measurement with ultrafast synchrotron X-ray imaging. The imaging rate of 1,000 frames per second (f.p.s. ), more than 15 times faster than that of conventional X-ray radiography (typically 30–60 f.p.s.) in large volume presses, enables us to precisely determine very low viscosity values. We find that viscosities of calcite and dolomite melts are surprisingly low, in the range of 0.006–0.010 Pa s, which are 1–3 orders of magnitude lower than those determined in previous experiment [26] and calculation [29] . These viscosities are so low that they are more similar to water [30] than to silicate melts [20] . Gravity-driven melt transportation (that is, without considering effects of shear deformation) is proportional to ‘hydrostatic melt mobility’, Δ ρ/η , where η is the viscosity of the melt and Δ ρ is density contrast between the melt and the surrounding solid rock, in addition to the permeability of the rock [20] , [31] , [32] . We find that the mobility of carbonate melts is ~2–3 orders of magnitude higher than that of basalt melts [20] . Highly mobile carbonate melts should play an important role in several magmatic processes in the Earth’s upper mantle, such as fast melt migration and effective melt extraction underneath mid-ocean ridges. Falling-sphere viscosity measurement by ultrafast imaging High-pressure viscosity measurements were conducted using a Paris–Edinburgh cell installed at Beamline 16-BM-B, HPCAT, at the Advanced Photon Source ( Supplementary Fig. 1 ). Falling velocity of the probing sphere was measured by ultrafast X-ray radiography using a high-speed camera with a 1,000 f.p.s. recording rate (exposure time of 1 ms). Supplementary Movie 1 shows a representative example of a falling Pt sphere in dolomite melt at 3.0 GPa and ~1,410 °C, in real time. Supplementary Movie 2 is the same movie but at a speed that is five times slower. 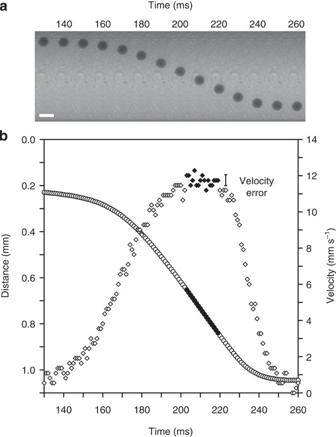Figure 1: Falling-sphere viscosity measurement using ultrafast X-ray imaging. (a) X-ray radiography images of falling Pt sphere (120 μm in diameter) in dolomite melt at 3.0 GPa and ~1,410 °C. Scale bar, 0.2 mm. (b) The results of the falling distance (open circles) and the falling velocity (open diamonds) for each frame (1 ms interval). Note that terminal velocity was achieved only at limited regions of falling distance (0.65–0.83 mm distance, indicated by filled symbols). The data clearly show that monitoring of the motion of falling sphere with substantial oversampling by using ultrafast imaging is essential to accurately determine terminal velocity and the resultant viscosity. Figure 1 shows a series of selected images of the Pt sphere at various times during the fall, as well as the sphere travel distance and speed as a function of elapsed time. The viscosity ( η ) was calculated with the Stokes equation including the correction factors for the effect of the wall ( F ) [33] and for the end effect ( E ) [34] : Figure 1: Falling-sphere viscosity measurement using ultrafast X-ray imaging. ( a ) X-ray radiography images of falling Pt sphere (120 μm in diameter) in dolomite melt at 3.0 GPa and ~1,410 °C. Scale bar, 0.2 mm. ( b ) The results of the falling distance (open circles) and the falling velocity (open diamonds) for each frame (1 ms interval). Note that terminal velocity was achieved only at limited regions of falling distance (0.65–0.83 mm distance, indicated by filled symbols). The data clearly show that monitoring of the motion of falling sphere with substantial oversampling by using ultrafast imaging is essential to accurately determine terminal velocity and the resultant viscosity. Full size image where v is the terminal velocity of the probing sphere, ρ and d are density and diameter, with subscripts s and l denoting properties of the probing spheres and liquid, respectively. Z is total height of the molten sample. With such a high-speed camera, the motion of the falling sphere could be monitored with substantial oversampling, enabling us to determine the terminal velocity accurately. Although the distance versus time plot ( Fig. 1b ) appears to show a large linear segment, careful analysis of the time derivatives shows that falling velocity reached a constant maximum (that is, terminal velocity: 11.6 mm s −1 ) within a rather limited region of the falling distance (0.65–0.83 mm), demonstrating that substantial oversampling is essential for terminal viscosity determination. It is difficult to measure this terminal velocity using the frame rates employed in previous falling-sphere viscosity measurements. To illustrate this, we simulated the falling-sphere image data with a reduced frame rate of 40 f.p.s., a typical frame rate used in previous experiments. At this frame rate, a maximum of four images are recorded at 25 ms per point ( Supplementary Fig. 2 ), with probing sphere falling distance forming an approximate straight line with elapsed time. Determining ‘terminal’ velocity through linear fitting of the falling distance data has been a commonly used methodology in previous viscosity studies. A linear fit to these four points yields a velocity (9.3 mm s −1 ), which is ~20% lower than that determined by high-speed imaging ( Supplementary Fig. 2 ), due to inappropriate sampling rate and analysis. The high frame rate used in the present study thus allows us to evaluate whether the sampling rate is sufficient to obtain a true constant velocity. Supplementary Fig. 3 shows a simulation of the falling velocity analyses with varying camera frame rates, by removing certain recorded images periodically. With decreasing camera frame rate, it becomes more difficult to define terminal velocity. At a frame rate of 250 f.p.s., it is possible to identify four data points with about the same falling velocity ( Supplementary Fig. 3b ). Below 100 f.p.s., however, no constant velocity region can be clearly determined ( Supplementary Fig. 3c–e ). Since between 250 and 1,000 f.p.s. we obtain identical values for the constant falling velocity, we conclude that terminal velocity has been reached in our experiments. Ultralow viscosity of carbonate melts Viscosity measurements were carried out up to 6.2 GPa at temperatures just above melting ( Supplementary Fig. 4 ), and the results are summarized in Table 1 . 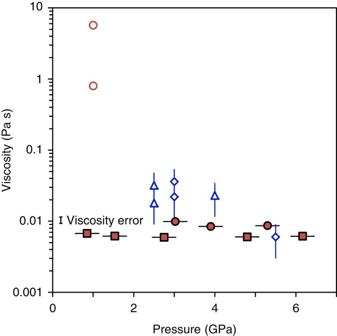Figure 2: Viscosities of calcite and dolomite melts. Viscosity measurements were carried out up to 6.2 GPa for calcite melts (solid dark red squares) and up to 5.3 GPa for dolomite melts (solid dark red circles) along the melting curves. Viscosities of a 70 wt.% CaCO3–30 wt.% MgCO3melt (open dark red circles) reported by previousex situfalling-sphere viscometry26and those of potassium carbonate (K2Mg(CO3)2(open blue diamonds) and K2Ca(CO3)2(open blue triangles)) melts27are shown for comparison. Error of our viscosity measurement (±9.3%) is much smaller than those in ref.27. Our obtained viscosity of calcite and dolomite melts are 2–3 orders of magnitude lower than those of previousex situviscosity measurements on a 70 wt.% CaCO3–30 wt.% MgCO3melt under 1 GPa (ref.26). Figure 2 shows viscosities of calcite and dolomite melts as a function of pressure along their respective melting curves [35] , [36] . For dolomite melts, viscosities were measured at pressures >2.9 GPa to avoid partial melting <~3 GPa (ref. 36 ). For both carbonate melts, ultralow viscosity values were obtained: 0.006–0.007 Pa s for calcite melt and 0.008–0.010 Pa s for dolomite melt. These low viscosities are more similar to those of water (for example, 0.001 Pa s at 1 atm and 20 °C; ref. 30 ) than those of silicate melts [20] , and are 2–3 orders of magnitude lower than those reported for a 70 wt.% CaCO 3 –30 wt.% MgCO 3 melt based on ex situ quench experiments (5.7 Pa s at 1,200 °C and 0.8 Pa s at 1,300 °C under 1 GPa; ref. 26 ). A calculation based on compiled molten salt data estimated a lower viscosity of 0.08 Pa s at 800 °C for CaCO 3 melt [29] . While this is about 1 order of magnitude higher than our results, comparison between the two studies is not straightforward because the temperature of the calculation (800 °C) is much lower than that of our experiments (1,380–1,790 °C) and below the melting temperature of CaCO 3 . The study by Dobson et al. [27] reported that viscosities of potassium carbonate (K 2 Mg(CO 3 ) 2 and K 2 Ca(CO 3 ) 2 ) melts are much lower than those of Ca–Mg carbonate melts [26] , [29] . Our viscosity results for CaCO 3 calcite and (Mg 0.40 Fe 0.09 Ca 0.51 )CO 3 dolomite melts are even 2–6 times lower than those of potassium carbonate melts at 2.5–4.0 GPa, and are similar to the lowest value obtained at 5.5 GPa in ref. 27 . However, experimental temperatures differ between this study (1,380–1,790 °C) and ref. 27 (800–1,200 °C). The viscosity difference may in part be due to this temperature contrast. Table 1 Experimental conditions and the viscosity results. Full size table Figure 2: Viscosities of calcite and dolomite melts. Viscosity measurements were carried out up to 6.2 GPa for calcite melts (solid dark red squares) and up to 5.3 GPa for dolomite melts (solid dark red circles) along the melting curves. Viscosities of a 70 wt.% CaCO 3 –30 wt.% MgCO 3 melt (open dark red circles) reported by previous ex situ falling-sphere viscometry [26] and those of potassium carbonate (K 2 Mg(CO 3 ) 2 (open blue diamonds) and K 2 Ca(CO 3 ) 2 (open blue triangles)) melts [27] are shown for comparison. Error of our viscosity measurement (±9.3%) is much smaller than those in ref. 27 . Our obtained viscosity of calcite and dolomite melts are 2–3 orders of magnitude lower than those of previous ex situ viscosity measurements on a 70 wt.% CaCO 3 –30 wt.% MgCO 3 melt under 1 GPa (ref. 26 ). Full size image Influence of temperature on viscosity of carbonate melts The above results show that calcite melt possesses lower viscosities than the dolomite melt. However, since we measured the viscosities of these melts along their respective melting curves, the effects of different melting temperatures may have contributed to the difference in measured viscosities. To separate the influences of temperature and composition, we conducted an experiment using a cell assembly with a double-layered probing sphere configuration ( Supplementary Fig. 1b ), which allowed us to control the temperature at which the probing sphere was released. We investigated the temperature dependence of the dolomite melt viscosity at a pressure of ~3 GPa. The results show that viscosity of dolomite melt is strongly temperature dependent ( Fig. 3 ). The temperature dependence of the viscosity of dolomite melt is similar to that of potassium carbonate melts [27] . In contrast, ref. 26 reported much stronger temperature dependence of viscosity for the 70 wt.% CaCO 3 –30 wt.% MgCO 3 melt than is seen in our results. 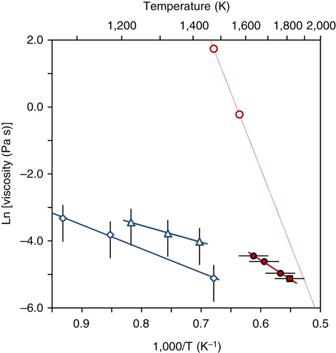Figure 3: Temperature dependence of viscosities of carbonate melts. The data in this study were obtained at ~3 GPa (2.8 GPa for CaCO3melt (solid dark red square) and 2.9 and 3.0 GPa for dolomite melt (solid dark red circles)) and are compared with previousex situviscosity measurements26(70 wt.% CaCO3+30 wt.% MgCO3) (open dark red circles) and those of potassium carbonate melts (K2Mg(CO3)2(open blue diamonds) and K2Ca(CO3)2(open blue triangles))27. Vertical and horizontal bars represent error of viscosity and temperature, respectively. Our data show a strong temperature dependence of the viscosity of the dolomite melt, which explains the viscosity difference between calcite and dolomite melts just above the melting temperatures. The data imply that there is almost no effect of composition on viscosity of calcite and dolomite melts. Figure 3: Temperature dependence of viscosities of carbonate melts. The data in this study were obtained at ~3 GPa (2.8 GPa for CaCO 3 melt (solid dark red square) and 2.9 and 3.0 GPa for dolomite melt (solid dark red circles)) and are compared with previous ex situ viscosity measurements [26] (70 wt.% CaCO 3 +30 wt.% MgCO 3 ) (open dark red circles) and those of potassium carbonate melts (K 2 Mg(CO 3 ) 2 (open blue diamonds) and K 2 Ca(CO 3 ) 2 (open blue triangles)) [27] . Vertical and horizontal bars represent error of viscosity and temperature, respectively. Our data show a strong temperature dependence of the viscosity of the dolomite melt, which explains the viscosity difference between calcite and dolomite melts just above the melting temperatures. The data imply that there is almost no effect of composition on viscosity of calcite and dolomite melts. Full size image Viscosities of dolomite and calcite melts fall on a single linear trend at ~3 GPa (2.8 GPa for calcite melt, and 2.9 and 3.0 GPa for dolomite melts; Fig. 3 ). Although the temperature dependence of calcite melt viscosity is uncertain, the similarity in temperature dependence of viscosities in potassium magnesium and calcium carbonate melts (ref. 27 ) implies that the effect of magnesium–calcium composition on the temperature dependence of viscosity may be insignificant, and that calcite and dolomite melts possess similar temperature dependence of viscosity. The data therefore suggest that the viscosity difference between calcite and dolomite just above the melting temperature is mainly attributable to different temperature conditions, and the effect of composition on the viscosity of calcite and dolomite melts may be negligible. Even after taking the influence of temperature into account, our measured viscosities of calcite and dolomite melts are much lower than those of previous ex situ viscosity measurements for 70 wt.% CaCO 3 and 30 wt.% MgCO 3 (ref. 26 ). Viscosities of both calcite and dolomite melts are essentially constant at high pressures at their respective melting temperatures [35] , [36] . This observation is consistent with the hypothesis by Poirier [37] , which suggests that viscosities of liquid metals can be scaled to the absolute melting temperature and that viscosities are constant along the melting curve with increasing pressure. We investigated the structure of the calcite and dolomite melts for each sample just after the viscosity measurement using the multi-angle energy dispersive X-ray diffraction technique [38] ( Fig. 4 ). These diffraction data show that cation–oxygen and cation–cation distances of the calcite melt up to 6.2 GPa and dolomite melt up to 5.3 GPa are constant with increasing pressure along their melting curves, implying that there are no structural changes in these melts within our pressure and temperature range. This is likely the physical origin of constant viscosities for these melts along their melting curves. 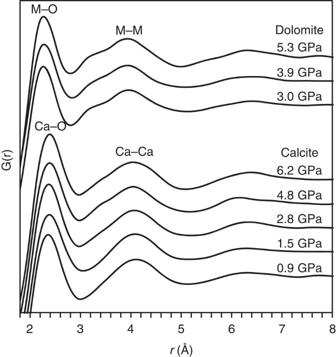Figure 4: Structure of calcite and dolomite melts at high pressures. The reduced pair distribution function G(r) was measured using the multi-angle energy dispersive X-ray diffraction technique38. A molecular dynamics simulation of calcite melt showed that Ca–O and Ca–Ca distances of calcite melt at 0.06 GPa and 1,327 °C is 2.327 Å and 4.173 Å, respectively (ref.41). We observed similar peak positions for calcite melt that are almost constant at pressures up to 6.2 GPa along the melting curve. In contrast, the first and second peaks of dolomite melts, which represent M–O and M–M distances (M=Ca, Mg and Fe), respectively, indicate slightly shorter distances than those of calcite melts. Similarly to the calcite melt, M–O and M–M distances of dolomite melts also showed almost constant values up to 5.3 GPa along melting temperatures. These data imply little structural change in the calcite and dolomite melts up to 6.2 GPa along the melting temperatures. Figure 4: Structure of calcite and dolomite melts at high pressures. The reduced pair distribution function G(r) was measured using the multi-angle energy dispersive X-ray diffraction technique [38] . A molecular dynamics simulation of calcite melt showed that Ca–O and Ca–Ca distances of calcite melt at 0.06 GPa and 1,327 °C is 2.327 Å and 4.173 Å, respectively (ref. 41 ). We observed similar peak positions for calcite melt that are almost constant at pressures up to 6.2 GPa along the melting curve. In contrast, the first and second peaks of dolomite melts, which represent M–O and M–M distances (M=Ca, Mg and Fe), respectively, indicate slightly shorter distances than those of calcite melts. Similarly to the calcite melt, M–O and M–M distances of dolomite melts also showed almost constant values up to 5.3 GPa along melting temperatures. These data imply little structural change in the calcite and dolomite melts up to 6.2 GPa along the melting temperatures. Full size image In addition, we find almost no compositional dependence in the viscosity between calcite (CaCO 3 ) and dolomite melts ((Mg 0.40 Fe 0.09 Ca 0.51 )CO 3 ). This is in contrast to the viscosity difference between K 2 Mg(CO 3 ) 2 and K 2 Ca(CO 3 ) 2 melts ( Fig. 3 ) noted by Dobson et al. [27] , who suggested a decrease in viscosity with increasing magnesium content). However, it is difficult to assess the claimed compositional effect due to the large uncertainties in their viscosity measurements ( Fig. 3 ). In fact, reported viscosity values of K 2 Mg(CO 3 ) 2 and K 2 Ca(CO 3 ) 2 carbonate melts are within the errors at 800–1,150 °C and 2.5–4.0 GPa, and only the data point of K 2 Mg(CO 3 ) 2 obtained at 5.5 GPa and 1,200 °C showed slightly lower viscosity than the other measurements ( Fig. 3 ). K 2 Mg(CO 3 ) 2 is unique among all carbonates in forming glass upon quenching [28] , which may explain the discrepancy in viscosity between K 2 Mg(CO 3 ) 2 and K 2 Ca(CO 3 ) 2 carbonate melts. 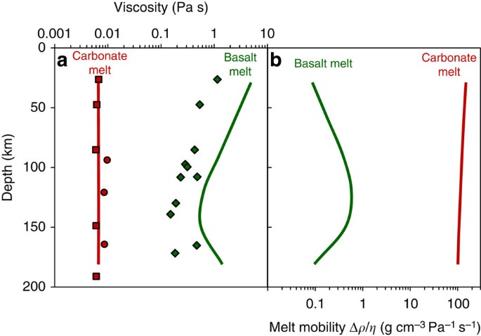Figure 5: Viscosity and mobility of carbonate and basalt melts. (a) Viscosities of carbonate melts at high pressures along their melting temperatures (1,380–1,790 °C) (dark red symbols) compared with those of basalt melts at 1,577 and 1,827 °C (dark green diamonds: ref.20). The dark red and dark green lines represent viscosities of carbonate and basalt20melts, respectively, along a geotherm39. (b) Mobility (Δρ/η) of carbonate and basalt melts20. Δρandηare density contrast between solid rock and melt and melt viscosity, respectively. The mobility of carbonate melt was calculated by using viscosity determined in this study and density of calcite from molecular dynamics simulation41with density of Fo90 (ref.40) as solid rock. Same parameters were used in the calculation of the mobility of basalt melt in ref.20. Figure 5a shows a comparison of viscosities of carbonates (calcite and dolomite) melts determined in this study and those of basalt melts reported in a previous study [20] at high pressures. To estimate viscosity of carbonate melts along a geotherm [39] , we fit our viscosity data for both calcite and dolomite melts to a function of pressure ( P , in GPa) and temperature ( T , in Kelvin) ( , where η 0 and T 0 are viscosity and temperature, respectively, at a reference condition, R is the gas constant, and A and B are fitting coefficients) [19] . Since there is little composition effect on the viscosity of calcite and dolomite melts, we fit both data together, to represent viscosities of (Ca,Mg±Fe)CO 3 melts. We obtained parameters of η 0 =0.0045 Pa s, T 0 =1,522 K, A =305 and B =179 with a s.d. of 0.0007 Pa s. Our obtained viscosity of carbonate melt is ~90–720 times lower than that of the basalt melt [20] at 1–6 GPa along an adiabatic geotherm [39] ( Fig. 5a ). The marked difference in viscosity between carbonate and basalt melts should yield a significant difference in the migration behaviour of these melts in the upper mantle. Figure 5: Viscosity and mobility of carbonate and basalt melts. ( a ) Viscosities of carbonate melts at high pressures along their melting temperatures (1,380–1,790 °C) (dark red symbols) compared with those of basalt melts at 1,577 and 1,827 °C (dark green diamonds: ref. 20 ). The dark red and dark green lines represent viscosities of carbonate and basalt [20] melts, respectively, along a geotherm [39] . ( b ) Mobility (Δ ρ/η ) of carbonate and basalt melts [20] . Δ ρ and η are density contrast between solid rock and melt and melt viscosity, respectively. The mobility of carbonate melt was calculated by using viscosity determined in this study and density of calcite from molecular dynamics simulation [41] with density of Fo90 (ref. 40 ) as solid rock. Same parameters were used in the calculation of the mobility of basalt melt in ref. 20 . Full size image Gravity-driven melt transportation is proportional to hydrostatic melt mobility, Δ ρ/η , where η is the viscosity of the melt and Δ ρ is density contrast between the melt and the surrounding solid rock, in addition to the permeability of the rock [20] , [31] , [32] . The study by Sakamaki et al. [20] discussed the mobility of the basalt melt in the upper mantle and showed that Δ ρ/η changes from 0.03 to 0.58 g cm −3 Pa −1 s −1 at 0–210 km depth. To compare the mobility of carbonate and basalt melts, we calculated the mobility of carbonate melts by adopting the same parameters as Sakamaki et al. [20] (adiabatic temperature gradient by Mckenzie and Bickle [39] , and density of Fo90 olivine by Circone and Agree [40] as density of solid rock). Densities of the calcite melt at various P – T conditions are based on results from molecular dynamics simulations [41] . Carbonate melts possess lower densities than basalt melts, further enhancing the contrast in melt mobility between basalt and carbonate melts beyond the significant differences in viscosity. As a result, the mobility of carbonate melts is 101–148 g cm −3 Pa −1 s −1 at 30–180 km depths, which is ~200–1,700 times higher than those of the basalt melt. The high mobility of carbonate melts has significant implications for magmatic processes in the Earth’s upper mantle. For example, melt segregation and magma focusing beneath mid-ocean ridges is an important magmatic process that may critically depend on carbonate melt migration. A fundamental geophysical observation of the mantle beneath mid-ocean ridges is that a low degree of melt is distributed over a broad region [42] , [43] . In addition, geochemical models of melting beneath mid-ocean ridges based on radioactive isotope disequilibrium predict that melt segregates from the matrix at very low porosities on the order of 0.1% and rises ~100 km in 1,600–8,000 years (melt ascent velocity of >10 m per year) (refs 44 , 45 ). These facts imply that small amounts of initially generated melts are efficiently extracted from the source region and transported towards the ridge axis to form the oceanic crust. However, because the basaltic melt has high-viscosity [20] with low mobility, high ascent velocity >10 m per year cannot be achieved by gravity-driven porous flow even by assuming the most favourable parameters for the basalt melt [46] . To efficiently extract and transport the highly viscous basaltic melt, several mechanisms, such as focused porous flow [47] , [48] , melt flow through open channel and/or fractures [49] , [50] and stress-driven melt segregation [51] , [52] , have been proposed. On the other hand, the high melt ascent velocity may simply be achieved with liquid of much lower viscosity than that of basalt melt, such as carbonate-rich melt. Faul [46] argued for the possibility of volatile-rich melts at the deeper part of the mid-ocean ridge to explain high melt ascent rate at low porosities, and recent experimental [10] and electrical conductivity [12] , [53] results suggest the existence of a small amount of carbonate-rich melt in the asthenosphere beneath the mid-ocean ridge. In addition, a geochemical study by Dasgupta et al. [54] suggested that the 230 Th and 231 Pa excesses observed in erupted mid-ocean ridge basalt are a consequence of contributions of carbonate-rich melt. These data suggest that, while basalts are erupted at mid-ocean ridges, the initial melts generated at depth in this environment may be carbonate rich, and that they progressively change to basaltic composition during ascent and melt-rock reaction [10] . We calculated the migration velocity of pure carbonate melts using the following equations [32] : where k is permeability, a is characteristic grain diameter, φ is melt fraction, n and C are numerical constants, g is the gravitational acceleration constant, and w 0 is the melt ascent velocity. We assumed a =2 mm and used n and C values of 2 and 1,600, respectively (according to the study by Bargen and Waff [55] ). Then, the melt ascent velocity was calculated for φ =0.001 with of carbonate melt obtained in this study (101–148 g cm −3 Pa −1 s −1 ). The calculation yielded a melt ascent velocity of ~80–115 m per year, which is higher than that constrained by radioactive isotope disequilibrium (>10 m per year) (refs 44 , 45 ). These data imply that the high mobility of pure carbonate melts can yield large enough migration velocities to satisfy constraints by radioactive isotope disequilibrium in the mantle deep beneath mid-ocean ridges. Carbonate-rich melts are likely to be strongly reactive with the silicate mantle during upward flow, leading to progressive change in the melt composition from carbonate rich to silicate rich with decreasing depth [10] . The CO 2 content of H 2 O-free carbonated peridotite melt decreases to ~20–25 wt.% upon rising to 150 km depth [10] , corresponding to a liquid with ca. 50 wt.% carbonate and 50 wt.% silicate. Significant changes in melt viscosity and melt-migration velocity should accompany this compositional evolution. However, the viscosity variation between carbonate and silicate melts is poorly understood, and studies of the effect of CO 2 on viscosity of silicate melts have considered only low CO 2 contents (up to 3.6 wt.%) [56] , [57] . To assess the influence of composition on the viscosity of carbonate-rich melts, we conducted preliminary experiments on CaCO 3 –CaSiO 3 melts using the same viscosity measurement technique. The results show that the logarithm of the viscosity of highly carbonated silicate melts displays a linear variation with composition across CaCO 3 and CaSiO 3 join ( Fig. 6 ). If carbonate–basalt melts are characterized by a viscosity-composition trend similar to that of CaCO 3 –CaSiO 3 melts, then carbonated silicate melt of 50 wt.% carbonate and 50 wt.% silicate at 150 km depth would possess viscosity ~9.5 times higher than pure carbonate melt, because the viscosity of carbonate melt along the geotherm is ~90 times lower than that of basalt melt [20] at 120–150 km depth ( Fig. 5 ). Although the ~9.5 times increase of viscosity may decrease melt-migration velocity proportionally, Dasgupta et al. [10] reported that the fraction of the melt increases by about a factor of 2 from ~0.025 wt.% at ~250 km depth to ~0.05 wt.% at ~150 km depth; this proportionally decreases melt-migration velocity according to equations (4) and (5). As a result, the migration velocity of the melt at ~150 km depth is only ~4–5 times lower than that of pure carbonate melt. It is important to note that while CaSiO 3 liquids contain a mixture of network forming SiO 2 and network modifying CaO, they are nevertheless a highly simplistic model for more complex silicate liquids such as basalt. Additional viscosity measurements on such liquids are necessary to refine these calculations. Nevertheless, our experiments imply that highly carbonated silicate melt could also migrate at speeds >10 m per year. 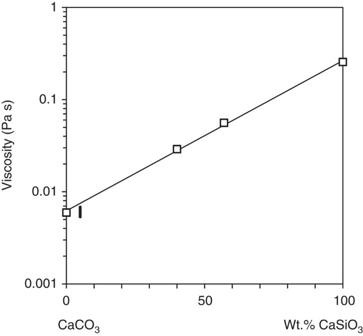Figure 6: Effect of composition between CaCO3and CaSiO3on melt viscosity. These mixtures display simple eutectic melting with no sub-solidus decarbonation reactions62, making them amenable to falling-sphere viscosity measurements. Viscosity measurements were conducted on 40, 57 and 100 wt.% CaSiO3at almost identical pressure (2.8–3.2 GPa) and temperature (1,500–1,570 °C) conditions. The thick vertical line represents variation of viscosity attributed to temperature variation between 1,500 and 1,570 °C estimated from temperature dependence of viscosity of carbonate melts inFig. 3. Viscosities of CaCO3–CaSiO3melts with 40 and 57 wt.% CaSiO3compositions lie on a linear line of Log10viscosity versus wt.% of CaSiO3between pure CaCO3and CaSiO3compositions. Figure 6: Effect of composition between CaCO 3 and CaSiO 3 on melt viscosity. These mixtures display simple eutectic melting with no sub-solidus decarbonation reactions [62] , making them amenable to falling-sphere viscosity measurements. Viscosity measurements were conducted on 40, 57 and 100 wt.% CaSiO 3 at almost identical pressure (2.8–3.2 GPa) and temperature (1,500–1,570 °C) conditions. The thick vertical line represents variation of viscosity attributed to temperature variation between 1,500 and 1,570 °C estimated from temperature dependence of viscosity of carbonate melts in Fig. 3 . Viscosities of CaCO 3 –CaSiO 3 melts with 40 and 57 wt.% CaSiO 3 compositions lie on a linear line of Log 10 viscosity versus wt.% of CaSiO 3 between pure CaCO 3 and CaSiO 3 compositions. Full size image High-pressure and high-temperature experiments Measurements were carried out in a standard Paris–Edinburgh cell assembly [38] with a cylindrical sample 1.5 mm in diameter and 1.6 mm in height enclosed in a graphite capsule ( Supplementary Fig. 1 ). The cell assembly mainly consists of a boron–epoxy gasket, MgO sleeve pressure medium, graphite heater and ZrO 2 thermal insulation cap. The ZrO 2 cap provides a good thermal insulator that reduces temperature variation in samples [58] . Temperatures were estimated by power–temperature relation curves that were determined in a separate experiment using an identical cell configuration [38] . The estimated temperatures were consistent with the melting curve of CaCO 3 (ref. 35 ) with a s.d. of 60 °C ( Supplementary Fig. 4 ). Reproducibility of the temperature calibration has been demonstrated previously [59] by reproducing the melting curves of NaCl and KCl with a s.d. of 50 °C at pressure conditions up to 7.3 GPa. The temperature gradient in the sample is uncertain, but the fact that a sphere placed at the top of the sample fell within 60 °C from the melting temperatures of CaCO 3 (ref. 35 ) implies that temperature gradient in the sample is not significant. Pressures were determined by the equation of state of MgO (ref. 60 ). Details of the Paris–Edinburgh cell high-pressure and high-temperature experiment are described elsewhere (ref. 38 ). Ultrafast X-ray imaging The ultrafast X-ray imaging was carried out using unfocused white X-rays with a beam size of 1.0 mm (horizontal) × 1.0–1.3 mm (vertical) depending on height of the PE cell at high pressures. We employed Ce-doped yttrium aluminium garnet (YAG:Ce) with a 45° mirror and a five times infinity-corrected objective lens (numerical aperture=0.14). Images were captured with a high-speed camera (Photron FASTCAM SA3). The pixel resolution of 5.46 μm per pixel was calibrated by using a WC ball with a 497 μm diameter. Falling-sphere viscosity measurement Falling-sphere viscosity measurements used Pt balls with diameters ranging from 84–153 μm as probing spheres ( Table 1 ). We analyzed the position of the Pt sphere in each frame by using the Tracker plugin in the ImageJ software package. The diameter of the Pt spheres was measured by X-ray radiography using a high-resolution camera with a pixel size of 0.95 μm per pixel (ref. 38 ). The density of the Pt spheres was calculated by the equation of state for platinum [61] . We used density information for the calcite melt reported by molecular dynamics simulations [41] . Unfortunately, the density of dolomite melt is not well-known. We therefore adopted the same density as the calcite melt in the dolomite viscosity calculation. The assumption does not significantly influence the viscosity determination because of the large difference in densities between Pt (for example, 21.45 g cm −3 at ambient condition) and the carbonate melts (2.2–2.6 g cm −3 ). For example, a 10% difference in the dolomite melt density would only change the viscosity by 1.3%. In contrast, it is known that the uncertainties in terminal velocity dominate the precision of the viscosity determination. In this study, terminal velocities were accurately determined with s.d. of ±1.4–3.9%. In addition, the uncertainty in the diameter of the probing sphere also contributes to errors in viscosity due to the small sphere size. Our high-resolution X-ray radiography has a ±2 μm resolution in imaging [38] , which causes ±2.1–4.1% uncertainty in viscosity. Therefore, the overall uncertainty in our viscosity determination is <±9.3%. How to cite this article : Kono, Y. et al. Ultralow viscosity of carbonate melts at high pressures. Nat. Commun. 5:5091 doi: 10.1038/ncomms6091 (2014).